Spatial fluctuations in barrier height at the graphene–silicon carbide Schottky junction When graphene is interfaced with a semiconductor, a Schottky contact forms with rectifying properties. Graphene, however, is also susceptible to the formation of ripples upon making contact with another material. Here we report intrinsic ripple- and electric field-induced effects at the graphene semiconductor Schottky junction, by comparing chemical vapour-deposited graphene transferred on semiconductor surfaces of opposite polarization—the hydrogen-terminated silicon and carbon faces of hexagonal silicon carbide. Using scanning tunnelling microscopy/spectroscopy and first-principles calculations, we show the formation of a narrow Schottky dipole barrier approximately 10 Å wide, which facilitates the observed effective electric field control of the Schottky barrier height. We further find atomic-scale spatial fluctuations in the Schottky barrier that directly follow the undulation of ripples on both graphene–silicon carbide junctions. These findings reveal fundamental properties of the graphene/semiconductor Schottky junction—a key component of vertical graphene devices that offer functionalities unattainable in planar device architecture. Graphene, one atomic layer of sp 2 -bonded carbon atoms that are closely packed in a honeycomb crystal lattice, is a semimetal with linearly dispersing states at low carrier energies [1] . When interfaced with semiconductors, Schottky barriers are formed at the graphene/semiconductor junctions with rectifying properties [2] that enable applications such as solar cells [3] , photodetectors [4] , Schottky diodes [5] and, most notably, three-terminal transistors with 10 6 on/off ratio [6] , [7] , facilitated by the effective tuning of the Schottky barrier height by an electric field. Graphene, however, is also prone to deformation in the direction normal to its surface, that is, the formation of ripples [8] , [9] , [10] , [11] when in contact with another material, or when placed under an applied electric field [12] , [13] . As these ripples are expected to modulate graphene’s electronic properties [14] , [15] , [16] , one critical question is whether they will have an impact on the Schottky barrier formation at the graphene/semiconductor junction. Here by comparing chemical vapour-deposited (CVD) graphene transferred on semiconductor surfaces of opposite polarization—the hydrogen-terminated 6H-SiC(0001) (Si face) and 4H-SiC(000 ) (C face)—we find that graphene ripples lead to spatial inhomogeneities in the Schottky barrier height. In addition, the large polarizability of graphene π states also leads to the formation of a narrow Schottky dipole barrier as high as 1.3 eV, but only ~10 Å wide, which is highly tunable by an electric field. These results provide insights into the fundamental properties of graphene/semiconductor Schottky junctions that enable the novel functionalities in vertical graphene devices [6] , [7] . Band alignment of graphene and H-terminated silicon carbide Graphene/semiconductor Schottky contacts are unlike their metal/semiconductor counterparts [17] , largely because of the tunability of the graphene work function [18] and the polarizability of the graphene π orbits at the junction by an electric field [1] . For graphene, the work function Φ G is defined by its Fermi level, which is at the Dirac point, E D . Thus, the relative values of Φ G and the semiconductor work function Φ S (referenced to the Fermi level for doped semiconductors) will determine whether graphene is effectively P- like ( Φ G < Φ S ) or n -like ( Φ G > Φ S ). For the polar semiconductor SiC studied here, both possibilities occur. To first order, the barrier height is given simply by the work function difference or, equivalently for intrinsic semiconductors, the difference between E D of graphene and the valence band maximum ( E VBM ) of SiC, as shown in Fig. 1 . For an interacting system, the barrier will be modified by the interface ‘Schottky dipole’ arising from the charge rearrangements at the junction [19] . As we show below, this is of particular significance for graphene because of the large polarizability of the π orbits by an electric field, either external or because of the surface dipole of the semiconductor. 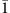Figure 1: Band alignment of graphene and H-terminated 6Η-SiC(0001) and (000). The calculated work functions for the H-terminated 6H-SiC(0001) (Si face) and 6H-SiC(000) (C face) are 6.09 and 3.98 eV, respectively. The work function difference between the Si and C faces is because of the polar nature of 6Η-SiC. The 5.13-eV value for graphene is obtained with a lattice constant (2.66 Å) matching the SiC substrate (compared with 4.54 eV for the equilibrium lattice constant of 2.46 Å) and gives estimated Schottky barriers of 0.96 eV for Si-face- and 1.15 eV for C-face junctions. (For the 4H polytype, with its larger bulk polarization, the simple estimates give 1.00 and 1.27 eV, respectively.) Figure 1: Band alignment of graphene and H-terminated 6Η-SiC(0001) and (000 ). The calculated work functions for the H-terminated 6H-SiC(0001) (Si face) and 6H-SiC(000 ) (C face) are 6.09 and 3.98 eV, respectively. The work function difference between the Si and C faces is because of the polar nature of 6Η-SiC. The 5.13-eV value for graphene is obtained with a lattice constant (2.66 Å) matching the SiC substrate (compared with 4.54 eV for the equilibrium lattice constant of 2.46 Å) and gives estimated Schottky barriers of 0.96 eV for Si-face- and 1.15 eV for C-face junctions. (For the 4H polytype, with its larger bulk polarization, the simple estimates give 1.00 and 1.27 eV, respectively.) Full size image Topology of SiC substrates Our experiments are carried out on CVD graphene transferred [20] on substrates of opposite polarization—6H-SiC(0001) and 4H-SiC(000 ). As revealed by atomic force microscopy (AFM), the as-received SiC substrates exhibit scratches tens of nm in depth because of polishing damages ( Fig. 2a ). Hydrogen etching at 1,600 °C removes these damages [21] and results in a step terrace morphology, with nominal step height of three or six Si-C bilayers and terraces of ~0.45 μm ( Fig. 2b ). This processing additionally leads to a chemically inert surface likely terminated with hydrogen or silicates [22] , [23] , which protects the SiC surface from oxidation during the transfer of graphene. 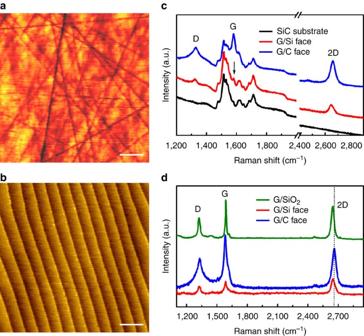Figure 2: Topography of SiC substrate and Raman spectra of transferred graphene. AFM images of the 6H-SiC(0001) substrate (a) before and (b) after the H2etching at 1,600 °C. The scale bars are 1 μm. The average step height inbis 1.4 nm (corresponding to approximately six Si-C bilayers) and the terrace size is 0.45 μm. (c) Raman spectra of the SiC substrate and graphene transferred on the Si and C faces. (d) Raman spectra of graphene on SiO2/Si and the Si and C faces of SiC after subtracting baselines and substrate contributions. Figure 2: Topography of SiC substrate and Raman spectra of transferred graphene. AFM images of the 6H-SiC(0001) substrate ( a ) before and ( b ) after the H 2 etching at 1,600 °C. The scale bars are 1 μm. The average step height in b is 1.4 nm (corresponding to approximately six Si-C bilayers) and the terrace size is 0.45 μm. ( c ) Raman spectra of the SiC substrate and graphene transferred on the Si and C faces. ( d ) Raman spectra of graphene on SiO 2 /Si and the Si and C faces of SiC after subtracting baselines and substrate contributions. Full size image Raman characterization of transferred grapheme Raman spectroscopy is used to confirm the transfer of graphene [24] . The spectrum of 6H-SiC(0001) has several features ( Fig. 2c ) between 1,400 and 1,800 cm −1 , attributed to optical phonons and transverse optical phonon replica [25] . The transferred graphene exhibits three additional peaks, which can be more clearly seen in the substrate–subtracted spectra ( Fig. 2d ). These peaks, located at 1,326, 1,582 and 2,655 cm −1 , are attributed to the defect-induced D band, the in-plane vibrational G band and the 2D band arising from double-resonant Raman scattering process, respectively [26] . The G and 2D bands of graphene on both the Si and C faces exhibit approximately the same frequencies, indicating that they are under similar stress [27] . The 2D bands are shifted ~10 cm −1 towards higher wave number compared with graphene on SiO 2 /Si, with full-widths at half-maximum of 40 and 42 cm −1 for the Si and C faces, respectively, consistent with single-layer graphene. The intensity ratio of the 2D to G peaks ( I 2D / I G =0.8) is less than one, a signature of doping in graphene [28] . In addition, the presence of the D band at ~1,326 cm −1 in both cases indicates the presence of residual defects in the graphene. Scanning tunnelling microcopy of graphene/H-SiC The surface morphology of transferred graphene on SiC is further characterized using scanning tunnelling microscopy (STM), as shown in Fig. 3a . Clearly evident is a distinct network of ridges 2.7±0.6 nm in height, 23.4±4.7 nm in width and hundreds of nm in length across the terraces where the underlying SiC substrate steps are still visible. These ridges are bulged regions of graphene [29] , [30] , originated from the CVD growth and preserved during transfer. 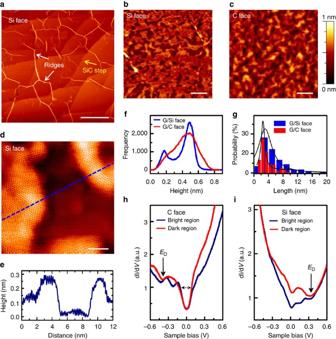Figure 3: Topography and dI/dVtunnelling spectra of graphene/H-SiC. (a) Large-scale STM image (500 nm scale bar) of graphene transferred on Si face SiC showing graphene ridges and underneath SiC steps (It=0.11 nA,Vs=−0.17 V). (b,c) Morphology of graphene on the Si face (It=0.1 nA,Vs=−0.05 V) and the C face SiC (It=0.1 nA,Vs=−0.17 V). The scale bars are 20 nm. (d) Atomic resolution image of dark and bright regions of graphene on the Si face (It=0.4 nA,Vs=−0.02 V, 2 nm scale bar). (e) Line profile along the dotted blue line ind. (f) Histograms of the measured heights of graphene on both the Si and C faces. The average separation between the maxima and minima of the ripples is ~0.33 nm for both faces. (g) Distribution of the width of the ripples (measured by width of the dark regions) for graphene on both faces, fitted to Lorentzian line shapes (solid lines). (h,i) dI/dVspectra of graphene transferred on the C and Si faces of SiC, respectively. Figure 3: Topography and d I /d V tunnelling spectra of graphene/H-SiC. ( a ) Large-scale STM image (500 nm scale bar) of graphene transferred on Si face SiC showing graphene ridges and underneath SiC steps ( I t =0.11 nA, V s =−0.17 V). ( b , c ) Morphology of graphene on the Si face ( I t =0.1 nA, V s =−0.05 V) and the C face SiC ( I t =0.1 nA, V s =−0.17 V). The scale bars are 20 nm. ( d ) Atomic resolution image of dark and bright regions of graphene on the Si face ( I t =0.4 nA, V s =−0.02 V, 2 nm scale bar). ( e ) Line profile along the dotted blue line in d . ( f ) Histograms of the measured heights of graphene on both the Si and C faces. The average separation between the maxima and minima of the ripples is ~0.33 nm for both faces. ( g ) Distribution of the width of the ripples (measured by width of the dark regions) for graphene on both faces, fitted to Lorentzian line shapes (solid lines). ( h , i ) d I /d V spectra of graphene transferred on the C and Si faces of SiC, respectively. Full size image Additional smaller spatial fluctuations (that is, ripples) are also observed between these ridges as shown in Fig. 3b,c for graphene transferred on the Si and C faces, respectively. Whereas the graphene honeycomb lattice is clearly continuous throughout the corrugations ( Fig. 3d ), analysis of line profiles ( Fig. 3e ) further indicates that the dark areas are likely in contact with the underlying SiC substrate, while the bright regions are buckled up from it, resulting in a warped graphene layer. An average ripple height of 0.33 nm is found for graphene on both substrates ( Fig. 3f ). Similarly, the lateral length scale (measured by the width of the dark region) is found to be 2.5 and 3.1 nm for graphene on the C and Si face, respectively ( Fig. 3g ). These results are similar to earlier STM studies of exfoliated graphene transferred on SiO 2/ Si [9] , [10] , [11] , suggesting that formation of ripples is universal for graphene transferred on a substrate, independent of whether the substrate is semiconducting or dielectric. Tunnelling spectroscopy of graphene/H-SiC The electronic properties of the transferred graphene/SiC are further investigated using scanning tunnelling spectroscopy (STS). On the C face, all spectra exhibit a gap of ~130 meV at zero bias ( Fig. 3h ), attributed to phonon-assisted tunnelling [31] . For the dark region, a local minimum at −0.39 eV is also evident, attributed to the Dirac point [31] . For the bright region, E D is shifted to −0.42 eV, whereas an additional dip at −0.23 eV also appears. On the Si face, qualitatively similar line shapes are also observed ( Fig. 3i ), with the minimum at 0.35 eV identified as E D , and an additional dip at +0.15 eV for the bright region. These results indicate that graphene transferred on C and Si faces of SiC are n- and p-type, respectively. To further illustrate the impact of ripples on the Dirac states, Fig. 4a shows spatially resolved dI/dV spectra taken on graphene/C face across a ripple at positions marked in Fig. 4b . All spectra exhibit the phonon gap, however, with variations in the Dirac point. Atop the bright region (spectrum 1 ), two strong peaks separated by ~0.23 eV (marked by up-pointing arrows) are observed, with their separation becoming progressively smaller towards the centre of the dark region, where only a broad peak at −0.24 eV is seen (spectrum 9 ). These two peaks re-emerge as the tip is moved towards the bright region (spectra 10 – 12 ). Similar behaviour is also observed for graphene/Si face ( Fig. 4c,d ). These observations clearly show that the spatial variations of E D directly follow the undulation of the ripples, with Gaussian distributions of full-width at half-maximum of 42 and 51 meV for graphene on the C face and Si face of SiC, respectively. These results are in direct contrast to the case for graphene on SiO 2 /Si substrate, where variations in E D are attributed to charge impurities in the SiO 2 substrate [9] , [10] , [11] , and not topographic fluctuations. The origin of the two additional peaks is unclear at the present, and are tentatively attributed to either additional states arising from quantum confinement in the buckled-up regions [32] , [33] , or mid-gap states in curved graphene [14] , [15] , [16] . 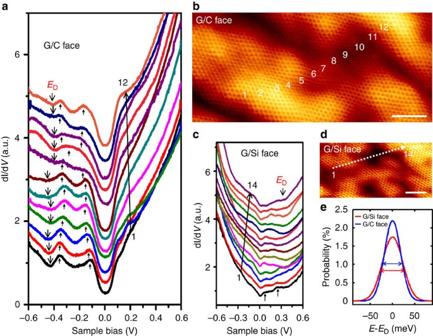Figure 4: Spatially resolved dI/dVtunnelling spectra of graphene/H-SiC. (a) dI/dVspectra taken at the positions marked inb, the STM image of graphene on C-face SiC (It=1.6 nA,Vs=−0.4 V, 2.1 nm scale bar). (c) dI/dVspectra taken at the positions marked ind, the STM image of graphene on the Si-face SiC (It=0.6 nA,Vs=−0.2 V, 1.6 nm scale bar). (e) Histograms of the variation of the Dirac point for graphene on the C and Si faces of SiC with FWHM of 42 and 51 meV, respectively. Figure 4: Spatially resolved d I /d V tunnelling spectra of graphene/H-SiC. ( a ) d I /d V spectra taken at the positions marked in b , the STM image of graphene on C-face SiC ( I t =1.6 nA, V s =−0.4 V, 2.1 nm scale bar). ( c ) d I /d V spectra taken at the positions marked in d , the STM image of graphene on the Si-face SiC ( I t =0.6 nA, V s =−0.2 V, 1.6 nm scale bar). ( e ) Histograms of the variation of the Dirac point for graphene on the C and Si faces of SiC with FWHM of 42 and 51 meV, respectively. Full size image Density functional theory calculations To determine the origin of the spatial fluctuations in E D , and whether they are directly tied to the graphene ripples, we calculate the position of E D − E VBM —a direct measure of the Schottky barrier—as a function of the separation d between the graphene layer and the SiC substrate, as shown in Fig. 5a for the Si and C faces of 6H-SiC. An immediate observation is that the relative positions of E D relative to E VBM indicate that graphene is p-type on Si face and n-type on C face, as expected from their work function differences. In addition, the value of E D − E VBM strongly depends on d , consistent with the experimental observation that E D fluctuates with graphene ripples. The calculated Schottky barriers (≡ E D − E VBM ) at the equilibrium separations (indicated by dots in Fig. 5a ) are 0.78 and 0.49 eV for the Si and C faces, respectively. (For 4H-SiC, the value for the C face is approximately the same but increases by ~0.1 eV for the Si face.) 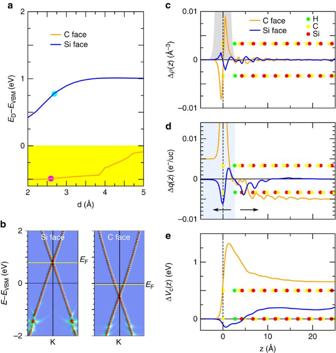Figure 5: Calculated bands, polarization, and potentials at the graphene/H-SiC junctions. (a) Calculated positions of the Dirac point relative to the VBM as a function of the separationdbetween graphene and the SiC surface; the solid dots denote the calculated equilibrium positions for 6H-SiC. (The calculations, even for larged, assume a common Fermi level, that is, the graphene and SiC are shorted. Thus,ED−EVBMfor largedis simply the calculated work function difference for the Si face, asEF=EDfalls in the SiC gap. For the C face, however,ED−EVBM→0; in the physical case where graphene and the substrate are uncoupled, this would also go to the work function difference, as inFig. 1. (b)k-projected bands around K of the 1 × 1 graphene Brillouin zone relative toEVBM. The calculated Fermi levels are also indicated. (c) Calculated planar-averaged electron polarization density perpendicular to the surface, Δρ(z), defined as the difference between the self-consistent electron densities of the combined system and the superposition of the isolated SiC substrate and graphene layers at the calculated equilibrium separations of the graphene and SiC substrate. The positions of the atomic layers are given by coloured dots, and the density for an isolated graphene layer is indicated by the solid grey region. (d) The integral of Δρ(z) per graphene unit cell, Δq(z), away from the interface for both graphene and SiC (with the arrows indicating the direction of integration); the solid light blue area indicates the graphene region. The maximum for the C face is 0.045 electron/unit cell. (e) Calculated Coulomb potentials corresponding to Δρ(z). Figure 5: Calculated bands, polarization, and potentials at the graphene/H-SiC junctions. ( a ) Calculated positions of the Dirac point relative to the VBM as a function of the separation d between graphene and the SiC surface; the solid dots denote the calculated equilibrium positions for 6H-SiC. (The calculations, even for large d , assume a common Fermi level, that is, the graphene and SiC are shorted. Thus, E D − E VBM for large d is simply the calculated work function difference for the Si face, as E F = E D falls in the SiC gap. For the C face, however, E D − E VBM →0; in the physical case where graphene and the substrate are uncoupled, this would also go to the work function difference, as in Fig. 1 . ( b ) k -projected bands around K of the 1 × 1 graphene Brillouin zone relative to E VBM . The calculated Fermi levels are also indicated. ( c ) Calculated planar-averaged electron polarization density perpendicular to the surface, Δ ρ ( z ), defined as the difference between the self-consistent electron densities of the combined system and the superposition of the isolated SiC substrate and graphene layers at the calculated equilibrium separations of the graphene and SiC substrate. The positions of the atomic layers are given by coloured dots, and the density for an isolated graphene layer is indicated by the solid grey region. ( d ) The integral of Δ ρ ( z ) per graphene unit cell, Δ q ( z ), away from the interface for both graphene and SiC (with the arrows indicating the direction of integration); the solid light blue area indicates the graphene region. The maximum for the C face is 0.045 electron/unit cell. ( e ) Calculated Coulomb potentials corresponding to Δ ρ ( z ). Full size image As the graphene Dirac states fall within a bulk SiC gap at the corresponding k values (plus the saturation of the dangling bonds by H), the k -projected graphene bands around the K point ( Fig. 5b ) for both faces are basically unaffected by interactions with the substrate SiC states—that is, graphene is a quasi-free-standing layer. For the Si face ( E D > E VBM ), no charge transfer is expected, as there are no unfilled SiC states below E D (= E F ) for electrons from graphene to flow into. That E F is at the Dirac point for the Si face is consistent with photoemission results obtained on hydrogen-intercalated epitaxial graphene on n-doped 6H-SiC(0001) [34] . For the C face, on the other hand, the Dirac point is below E VBM , so that states above E D are now occupied. The calculated E F for the whole system is ~0.03 eV below E VBM , indicating that there is a hole pocket in the vicinity of the interface. Next, the modification of the graphene Dirac states due to the electric field arising from the intrinsic surface dipole of the SiC substrate is calculated. The spatial distribution of the calculated planar-average polarization density Δ ρ ( z ) for the equilibrium graphene–substrate separations (that is, at the d values denoted by the dots in Fig. 5a ) is shown in Fig. 5c , along with the electron density from an isolated graphene layer for comparison. The polarization densities are opposite in sign on either sides of the graphene layer, giving rise to large polarization dipoles. In addition, the fact that Δ ρ ( z ) is both larger and of opposite sign for the C face compared with the Si face reflects the relative difference in E D versus E F for the two cases. This large polarization dipole formation in graphene, with Δ ρ ( z ) in the interface region orders of magnitude larger than the nominal bulk doping of ~10 18 cm −3 (10 −6 Å −3 ), is a direct consequence of the high polarizability of its π orbitals. Varying the graphene–substrate separation, d , alters the quantitative values of the polarization densities Δρ(z); however, the shapes and qualitative differences between the two faces remain. The integral of the polarization density Δ ρ ( z ) as a function of the distance away from the interface, Δ q ( z ) ( Fig. 5d ), provides a measure of charge transfer to/from graphene for both the graphene (shaded area) and the SiC substrate. (The interface is chosen to be at the H plane, rather than the more traditional midpoint between atomic layers so that the majority of the graphene density is in the ‘graphene’ region, cf ., Fig. 5c ) For the Si face, even though there is little or no overall charge transfer (that is, Δ q ~0 for z far outside the graphene), a region ~10 Å wide with a deficit of electrons (corresponding to a hole doping of ~5 × 10 12 cm −2 ) is formed as a result of an image dipole across the interface in the SiC. The graphene layer itself, except for a region just at the interface, is p-doped. Thus, whereas the coincidence of E F and E D indicates no charge transfer ( Fig. 5b ), the spatial distribution of the polarization suggests P -type doping of graphene, consistent with earlier transport measurements of H-intercalated epitaxial graphene/Si face [35] . For the C face, on the other hand, there is a charge transfer of ~0.005 electron per graphene cell (~10 13 cm −2 ), in good agreement with the calculated separation between E F and E D of ~0.45 eV ( Fig. 5b ), and thus transport measurements of graphene on the C face is expected to exhibit n-type behaviour. The charge transferred to graphene is mainly localized between the graphene and the substrate. To compensate the n-doping of the graphene Dirac states, the SiC has a narrow net p-doped region just beyond the first SiC bilayer, as a result of the n-like image dipole contribution and the p-doping from the image charge. These polarization densities Δ ρ ( z ) directly give rise to changes in the Coulomb potential, shown in Fig. 5e , and the differences between Δ V c (± ∞ ) is the Schottky dipole [19] . The spatial extent of the barriers in Δ V c is only ~10 Å, orders of magnitude smaller than the depletion regions in conventional metal–semiconductor systems [17] . The formation of these highly localized barriers is again a direct consequence of the large polarizability of the graphene π orbitals and points to opportunities for effectively tuning the barrier height by an applied field in graphene/semiconductor Schottky contacts. We note the importance of energy reference in comparing calculated and experimental results. In both the DFT calculations and photoemission experiments, E F is a natural zero separating occupied and unoccupied states, as evidenced by the excellent agreement between photoemission results and calculations for the Si face ( Fig. 5b ). For graphene/C face, tunnelling spectra give a barrier of 0.39±0.04 eV, in good agreement with the calculated value of 0.45 eV (no experimental photoemission or transport data on the C face are available for comparison). For graphene/Si face, on the other hand, whereas the Schottky barrier measured in transport studies (0.91 eV) [2] is close to the calculations (0.78 eV), tunnelling spectroscopy yields a smaller value of 0.35±0.05 eV ( Fig. 3i ). Tip-induced doping in STS [36] and uncertainties in the calculation of the polarizability arising from the choice of exchange-correlation potentials (among other calculation parameters) may contribute to the difference. Whereas the calculated Schottky barriers are referenced to the E VBM , the SiC substrates used in the experiments are n-type with the bulk Fermi level a few tenth of eV below the conduction band edge [22] . The use of E VBM as the reference is consistent with the freestanding nature of the transferred graphene and the Fermi level pinning within the SiC gap near the valence band edge [37] . This is further supported by the fact that the nominal bulk n-type doping of ~10 18 cm −3 (10 −6 Å −3 ) is orders of magnitude smaller than polarization densities at the graphene/SiC interface ( Fig. 4c ) and by the existence of a narrow p-doped layer near the interface in SiC for both Si and C faces. In summary, we find that intrinsic ripples form in graphene/H-SiC Schottky junctions, resulting in local inhomogeneities in the Schottky barrier height. The large polarizability of the graphene π states leads to the formation of a narrow Schottky dipole barrier that is highly tunable by electric field. For other (including non-polar) semiconductors, whether an image dipole forms or charge transfer occurs will depend on the position of E D (tunable by an external electrical field) relative to the bulk Fermi level of the semiconductor. This atomic-scale understanding of the fundamental properties of graphene/semiconductor Schottky contact will expedite to the development of vertical graphene devices with functionalities that are unattainable in planar device geometry [6] , [7] . Sample preparation Nitrogen-doped 6H-SiC(0001) and 4H-SiC(000 ) substrates (Cree, Inc.) are prepared by etching at 1,600 ° C in H 2 /Ar atmosphere for 15 min to remove polishing damages. This also results in a chemically inert surface likely terminated with hydrogen or silicates. CVD graphene (Graphene Supermarket) is transferred on these SiC substrates using standard polymethyl methacrylate (PMMA)-based technique. A post annealing in an Ar atmosphere at ~300 °C is performed to help remove residual photoresists. AFM and Raman and STM/STS measurements The as-received and hydrogen-etched SiC substrates are characterized by contact AFM in an ambient environment. Raman spectra are obtained using a 633-nm HeNe laser. STM imaging is carried out with electrochemically etched W tips or mechanically sharpened Pt tips at room temperature and liquid nitrogen temperature in ultrahigh vacuum with a base pressure <1 × 10 −10 Torr. The d I /d V tunnelling spectra are acquired by turning off the feedback loop and holding the tip at a fixed distance above the surface at liquid nitrogen temperature. A small a.c. modulation of 12 mV at 860 Hz is applied to the tip voltage, and the corresponding change in current is measured using lock-in detection. DFT calculations Density functional theory calculations are performed using the Vienna ab initio simulation package [38] in the projector-augmented wave framework. The exchange correlation functional is described by the general gradient approximation of Perdew–Burke–Ernzerhof [39] . The SiC(0001)–graphene systems are modeled using nine bilayers of ✓ 3 × ✓ 3 4H and 6H-SiC(0001) supercells (with an in-plane lattice constant of 3.073 Å) combined with 2 × 2 graphene layers and a vacuum region of 25 Å. Both sides of the slabs are terminated by H. To avoid artificial interactions between the polar slabs, two such slabs, oppositely oriented, are placed in each supercell, for a total of 136 atoms per cell. The outer several bilayers and graphene are fully relaxed for the minimum energy separation. With the H-termination, the graphene layers remain intact and approximately planar. The plotted bands are both spatially weighted and k -projected. The difference densities are obtained from separate calculations with the atomic positions of the atoms the same; the planar-averaged difference densities were then integrated numerically. How to cite this article: Rajput, S. et al. Spatial fluctuations in barrier height at the graphene–silicon carbide Schottky junction. Nat. Commun. 4:2752 doi: 10.1038/ncomms3752 (2013).